Charge density waves in the graphene sheets of the superconductor CaC6 Graphitic systems have an electronic structure that can be readily manipulated through electrostatic or chemical doping, resulting in a rich variety of electronic ground states. Here we report the first observation and characterization of electronic stripes in the highly electron-doped graphitic superconductor, CaC 6 , by scanning tunnelling microscopy and spectroscopy. The stripes correspond to a charge density wave with a period three times that of the Ca superlattice. Although the positions of the Ca intercalants are modulated, no displacements of the carbon lattice are detected, indicating that the graphene sheets host the ideal charge density wave. This provides an exceptionally simple material—graphene—as a starting point for understanding the relation between stripes and superconductivity. Furthermore, our experiments suggest a strategy to search for superconductivity in graphene, namely in the vicinity of striped 'Wigner crystal' phases, where some of the electrons crystallize to form a superlattice. Graphene, the archetypal two-dimensional (2D) material, has a unique electronic structure that can be significantly modified not only when cut, folded or rolled [1] , but also when assembled with dopant layers between graphene sheets to form graphite intercalation compounds [2] . The ground states of graphitic materials can be metallic, semi-metallic or semiconducting, depending on the allotrope form or intercalated species, and some have even been shown to superconduct [2] , [3] with transition temperatures ( T c ) above 10 K (ref. 4 , 5 ). Charge density waves (CDWs) are a symmetry-reducing ground-state most commonly found in layered materials [6] . Many such materials, including the transition-metal dichalcogenides [7] , [8] , [9] , metal-containing organic compounds [10] , and cuprate high-temperature superconductors [11] , exhibit superconductivity as well as CDWs [12] , [13] . It is, therefore, very natural to ask whether graphene, the simplest 2D material, can host a CDW/striped state [1] , [2] , [14] . The most obvious and direct method to search for such a state is to introduce carriers through a field-effect gate, and then to measure the properties using electrical, thermodynamic and local probes such as scanning tunnelling microscopy (STM) and spectroscopy (STS). There are already hints of insulating CDW states (in this case, referred to as 'Wigner crystals' in keeping with the nomenclature of semiconductor physics) for the highest carrier densities, of order 10 −3 electrons per carbon atom, which can be introduced with the field effect in suspended graphene [15] . The introduction of calcium atoms between graphene sheets ( Fig. 1a ) enables significantly greater electron doping of the graphite host and therefore provides a much better opportunity for STM and STS discoveries; ~0.2 electrons per carbon atom are donated to the graphitic π * band in CaC 6 (refs 16 , 17 ). Furthermore, the material is the optimum superconductor in its class with the highest known superconducting temperature ( T c =11.5 K) of any intercalated graphite [4] . 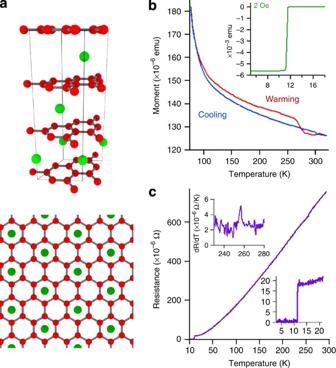Figure 1: The magnetization and transport properties of CaC6. (a) CaC6rhombohedral structure as measured by X-ray diffraction and 'expected STM view' of first graphene and Ca layers. Carbon atoms appear in red; Ca atoms appear in green. An unexpected transition occurs at high temperature in (b) the temperature-dependent DC magnetization at 1T and (c) temperature dependent four-contact resistance measurements. Inset in (b): superconducting transition with width ΔT~0.3 K. Inset in (c): superconducting transition, derivative of high-temperature transition. Inset units are the same as main figure unless otherwise stated. Figure 1: The magnetization and transport properties of CaC 6 . ( a ) CaC 6 rhombohedral structure as measured by X-ray diffraction and 'expected STM view' of first graphene and Ca layers. Carbon atoms appear in red; Ca atoms appear in green. An unexpected transition occurs at high temperature in ( b ) the temperature-dependent DC magnetization at 1T and ( c ) temperature dependent four-contact resistance measurements. Inset in ( b ): superconducting transition with width Δ T ~0.3 K. Inset in ( c ): superconducting transition, derivative of high-temperature transition. Inset units are the same as main figure unless otherwise stated. Full size image In this work, we use STM and STS to discover a striped CDW hosted by the graphene sheets of CaC 6 . Detailed topographic and spectroscopic measurements show a physical and electronic distortion of the superlattice and gapping of the local density of states (LDOS) associated with the CDW. Bulk transport measurements Figures 1b and c present DC magnetization, at a 1 T field parallel to the c -axis, and four-contact electrical transport measurements for a high-quality CaC 6 platelet (Methods). Insets in both figures demonstrate a sharp superconducting transition (Δ T ~0.3 K) at 11.5 K. Additionally, both techniques reveal an unexpected transition at ~250 K. The transition was reproducible on warming in three out of three samples at T CDW =250±10 K in magnetization, which is a thermodynamic bulk quantity. Cooling through T CDW yielded the blue curve in Figure 1b , for which the transition disappears. These data motivated a search for a corresponding effect in electrical transport, and we were able to identify a subtle transition in resistivity at 250±20 K in 5 out of 13 samples. In the CDW state the gapping of the Fermi surface (FS) typically leads to a reduction in the material conductivity. However, we report an enhancement of the metallic properties of CaC 6 in the CDW phase ( Fig. 1b,c ). Although this seems unusual, NbSe 2 , one of the most widely studied CDW systems [18] , [19] , [20] , displays a similar phenomenon. Furthermore, analogous effects have been seen in the high-temperature superconducting cuprates around the pseudogap temperature [21] , which some ascribe to a CDW transition [22] . Atomic resolution STM imaging STM is a versatile probe of CDWs, because it accesses structural information as well as the electronic spectrum, including—most notably—the CDW gap. We have employed the technique to determine the structure and electronic LDOS of CaC 6 at 78 K, above the superconducting transition but below the anomalous transition shown in Figure 1 . We report two surface types. The first matches the expected structure represented in Figure 1a : a hexagonal lattice ( a =0.250 nm), typical of STM-imaged graphite [23] or graphene [24] , superposed on a hexagonal Ca superlattice (0.433 nm=√3 a ) rotated by 30° (R30°) with respect to the primary lattice [25] . 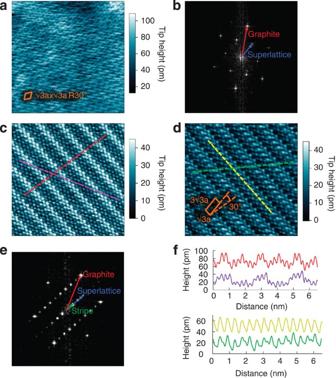Figure 2: Constant current STM images of CaC6surfaces recorded at 78 K. (a) Expected phase surface recorded at +300 mV matching the structure of CaC6as measured by X-ray diffraction. (b) Fourier transform of (a) displaying hexagonal carbon lattice (a=0.25 nm) with √3a×√3a 30° rotated Ca superlattice. (c) 7 nm×7 nm stripe phase surface with one-dimensional, 1.125 nm period, modulation recorded at +300 mV sample bias. (d) 7 nm×7 nm stripe phase surface at +400 mV (e) Fourier transform of (c) displaying both hexagonal structures as seen for the expected phase and the stripe that shares one of the Ca symmetry directions. (f) Line profiles in carbon symmetry directions as marked in (c) and in Ca symmetry directions as marked in (d). (a), (c) and (d) were recorded at 50 pA set point current. Unit cells for each surface type are shown in (a) and (d). This surface is referred to as the expected phase, and is shown in Figure 2a . The image presented was recorded at +300 mV sample bias, and it was found that varying the bias has no significant effect on the imaging of the expected phase. The graphite and superlattice periodicities are clearly visible in the Fourier transform image presented in Figure 2b . The principal finding of our experiment is a stripe phase, shown at, respectively, 300 mV and 400 mV sample bias in Figure 2c,d . The stripe phase, imaged under the same tunnelling conditions, on the same sample, has the underlying structure of the expected phase with an extra superposed long-range one-dimensional modulation. Figure 2: Constant current STM images of CaC 6 surfaces recorded at 78 K. ( a ) Expected phase surface recorded at +300 mV matching the structure of CaC 6 as measured by X-ray diffraction. ( b ) Fourier transform of ( a ) displaying hexagonal carbon lattice ( a =0.25 nm) with √3a×√3a 30° rotated Ca superlattice. ( c ) 7 nm×7 nm stripe phase surface with one-dimensional, 1.125 nm period, modulation recorded at +300 mV sample bias. ( d ) 7 nm×7 nm stripe phase surface at +400 mV ( e ) Fourier transform of ( c ) displaying both hexagonal structures as seen for the expected phase and the stripe that shares one of the Ca symmetry directions. ( f ) Line profiles in carbon symmetry directions as marked in ( c ) and in Ca symmetry directions as marked in ( d ). ( a ), ( c ) and ( d ) were recorded at 50 pA set point current. Unit cells for each surface type are shown in ( a ) and ( d ). Full size image The stripes have a periodicity of 1.125 nm and are commensurate with both the carbon and Ca lattices. The unit cell for the stripe phase is tripled in one of the Ca lattice directions. Consequently, the new unit cell is 3√3a×√3a R30° (1.299 nm×0.433 nm), as shown in Figure 2c,d . An amplitude plot of the Fourier transform of Figure 2c is shown in Figure 2e . The reciprocal lattice vectors for the stripe (blue), carbon (red) and Ca (green) lattices are marked on the image. The carbon and Ca lattice vectors correspond to the directions of the atomic planes indicated by the matching coloured lines seen in Figure 2c,d . The Ca atomic corrugation for the stripe phase is ~0.020 nm that is much lower than the X-ray-measured C–Ca distance of 0.226 nm (ref. 25 ) and the Ca 2+ ionic radius of 0.100 nm, indicating that the Ca atoms are subsurface and that the surface is graphene-terminated. Indeed, we found that high-resolution imaging of the stripe phase requires a high-purity sample and a large flat graphene-terminated surface. We believe non-graphene-terminated surfaces are not atomically resolvable owing to surface instability or roughness, which may also explain imaging difficulties reported by Bergeal et al . [26] Structural analysis The Ca superlattice is less prominent in real-space imaging at 300 mV ( Fig. 2c ) than it is at 400 mV ( Fig. 2e ), allowing us to analyse each lattice individually. Figure 2f displays line profiles taken along the carbon and Ca lattice symmetry directions, corresponding to the coloured lines marked in Figure 2c,d respectively. The profiles along the carbon lattice show no observable in-plane distortion from the ideal lattice configuration and no out-of-plane modulation of the atomic corrugation other than the stripe itself. Similarly, the Ca lattice exhibits no unexplained out-of-plane modulation. However, the profile taken in the Ca symmetry direction crossing the stripes (marked in green in the figure) shows some in-plane anomalies. Further analysis reveals the origin of these anomalies. 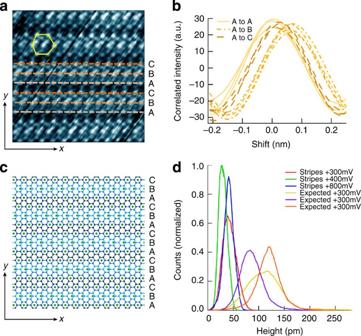Figure 3: Surface structure and the broken symmetry of the Ca superlattice. (a) 5 nm×5 nm drift-corrected topographic STM image with line profiles in the Ca-parallel-to-stripe symmetry direction marked on [B] and off [A, C] the stripe apex. (b) Correlation of line profiles shown in (a) demonstrate a 0.06±0.02 nm perturbation of the Ca atoms on the stripe apex. (c) A schematic illustrating the distortion of the Ca lattice (green) and the resultant stripe modulation (blue scale) on the graphene sheet as seen in positive sample bias imaging oriented to match (a). (d) Topographic height distributions for three different striped surface areas at a number of sample biases (as indicated in the legend) and three expected phase surface regions at +300 mV. Figure 3a is a drift-corrected (see Methods for details) version of Figure 2d . An overlay (shown in yellow in Fig. 3a ) connects a set of Ca atoms. The distortion of this overlay from the ideal hexagonal shape illustrates the perturbation of the Ca lattice from its ideal configuration. The perturbation is due to a systematic distortion of the Ca lattice whereby every third row of Ca atoms parallel to the stripes is shifted in the positive x -direction. To quantify this, we have labelled three distinct rows of Ca atoms ( Fig. 3a ): A, B and C which correspond to atoms below, coincident with and above the bright region of the stripe, respectively. By cross-correlating matching line profiles taken from these positions, as shown in Figure 3b , we find a 0.06±0.02 nm shift in the positive x -direction of the B Ca atoms, that is, those co-incident with the peak of the stripe, from their ideal lattice position with respect to the A and C atoms. Similar analysis did not reveal any distortion in the carbon lattice ( Supplementary Fig. S1 ). The distortion of the Ca lattice is an in-plane transverse wave only. Figure 3c is a schematic illustrating the new structure. The significant modulation of the Ca atomic positions is in sharp contrast to the lack of distortion we detect in the carbon lattice. However, we certainly cannot rule out modulations smaller than the in-plane instrumental resolution of 0.01 nm. Higher resolution momentum space techniques, such as X-ray or neutron scattering, could be used to detect smaller average modulations. Figure 3: Surface structure and the broken symmetry of the Ca superlattice. ( a ) 5 nm×5 nm drift-corrected topographic STM image with line profiles in the Ca-parallel-to-stripe symmetry direction marked on [B] and off [A, C] the stripe apex. ( b ) Correlation of line profiles shown in ( a ) demonstrate a 0.06±0.02 nm perturbation of the Ca atoms on the stripe apex. ( c ) A schematic illustrating the distortion of the Ca lattice (green) and the resultant stripe modulation (blue scale) on the graphene sheet as seen in positive sample bias imaging oriented to match ( a ). ( d ) Topographic height distributions for three different striped surface areas at a number of sample biases (as indicated in the legend) and three expected phase surface regions at +300 mV. Full size image The topographic height variations in Figure 2c,d are typical of the striped surface, whereas the expected surface had at least twice the total topographic variation as can be seen in Figure 2a . The difference in surface roughness between the two surface types is also evident from the height histograms presented in Figure 3d . Whereas the roughness of the stripe phase does not change significantly between different areas, the expected phase shows some variation for different surface regions. Also, the appearance of the stripe surface varies with bias (for example, Fig. 2c,d ), but this has a negligible effect on the surface roughness observed. For the two surfaces for which it was observed, the stripe phase eventually transformed into the expected phase. This was a one-way process and the stripe phase had a life span of 4–36 h. In the event of this transformation, STM resolution was lost for a short period (~5 min) after which the expected phase was resolved and the topographic height variation of the surface doubled. Filled and empty states The broken crystallographic symmetry of the Ca lattice is also reflected in the electronic behaviour of the Ca atoms, as observed in bias-dependent topographic imaging. 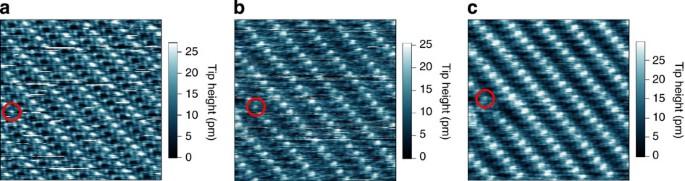Figure 4: Bias dependence of the stripe phase topography. 7 nm×7 nm constant current STM images of the CaC6stripe phase at (a)+600 mV, (b) +700 mV and (c) +800 mV sample bias. All three images were recorded at 50 pA tunnelling current at approximately the same surface location (a spatial reference point has been marked by a red circle in each image). Figure 4 shows that the topographic height of the perturbed superlattice position dominates the image above 600 mV, indicating a significantly greater density of unoccupied states at this position. 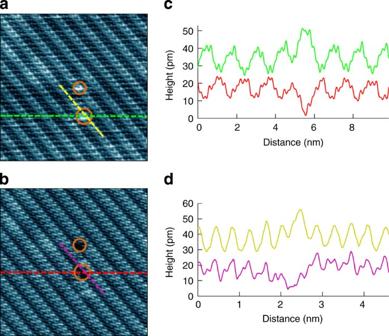Figure 5: Near perfect inversion of stripe contrast with bias polarity. Comparison of defect positions (circled) on 10 nm×10 nm topographic STM images recorded at (a) −700 mV and (b) +700 mV sample bias, demonstrate stripe modulation shiftsπout of phase with bias polarity change. (c) Line profiles marked in (a) (green) and (b) (red) demonstrate contrast inversion of defects and stripe modulation with change of bias polarity. (d) Line profiles marked in (a) (yellow) and (b) (purple) showing that Ca lattice contrast does not invert with bias. This can also be seen by comparing the lines marked in images (a) and (b) with the relative position of the stripe modulation. Both images were recorded at 50 pA tunnelling current. Figure 5 shows the behaviour of the stripes with bias inversion, as seen by topographic imaging at ±700 mV. The same two defects are circled in both images; at negative bias ( Fig. 5a ), the positions of both defects coincide with the peak of the stripe modulation and the Ca lattice is centred on the middle of the stripe troughs. At positive bias ( Fig. 5b ), the two defects coincide with the trough of the stripe modulation and the Ca lattice is centred on the middle of the stripe peaks. The stripe contrast inverts with change in bias polarity ( Fig. 5c ) while the Ca lattice contrast does not ( Fig. 5d ). The remarkable implication is that the stripe contrast involves only the electrons in the graphene planes. Figure 4: Bias dependence of the stripe phase topography. 7 nm×7 nm constant current STM images of the CaC 6 stripe phase at ( a) +600 mV, ( b ) +700 mV and ( c ) +800 mV sample bias. All three images were recorded at 50 pA tunnelling current at approximately the same surface location (a spatial reference point has been marked by a red circle in each image). Full size image Figure 5: Near perfect inversion of stripe contrast with bias polarity. Comparison of defect positions (circled) on 10 nm×10 nm topographic STM images recorded at ( a ) −700 mV and ( b ) +700 mV sample bias, demonstrate stripe modulation shifts π out of phase with bias polarity change. ( c ) Line profiles marked in ( a ) (green) and ( b ) (red) demonstrate contrast inversion of defects and stripe modulation with change of bias polarity. ( d ) Line profiles marked in ( a ) (yellow) and ( b ) (purple) showing that Ca lattice contrast does not invert with bias. This can also be seen by comparing the lines marked in images ( a ) and ( b ) with the relative position of the stripe modulation. Both images were recorded at 50 pA tunnelling current. Full size image Spectroscopic analysis To explore the electronic structure of the stripe phase in more detail we employed Current Imaging Tunnelling Spectroscopy (CITS). This technique yields a position-dependent current map, I( r ,V), where r is the position vector. The extracted current–voltage curves were numerically differentiated to access conductivity, g ( r ,V)=dI( r ,V)/dV, which is closely related to the LDOS [27] . 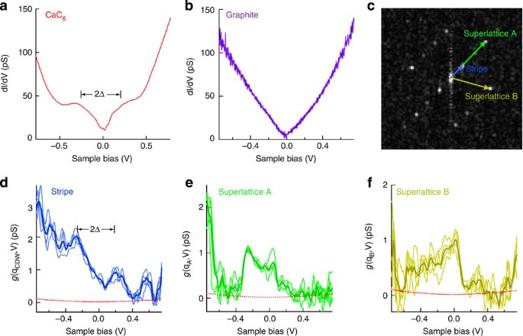Figure 6: Spectroscopic studies of stripe phase. (a) Numerically differentiated and averaged (60,000 spectra) spectroscopy,g(V) recorded at +800 mV, 50 pA set point on CaC6. (b) Numerically differentiated spectra recorded at the same set point on unintercalated graphite. (c)g(q,V) Fourier transform scanning tunnelling spectroscopic image at 0 mV. (d–f)g(q,V) Fourier intensity plotted as a function of energy for the stripe (d, blue) and Superlattices A and B (e, green and &f, yellow) spots marked in (b) respectively. These colours are chosen to match the respective directions marked inFigure 2. Faint lines represent individual datasets, bold lines represent average. Red dotted line is the background intensity (already subtracted from all lines presented). For the spatially averaged conductivity ( g (V)) of a striped CaC 6 surface, shown in Figure 6a , the most notable feature is a gap of 2Δ~475 mV at the Fermi level. The total zero bias conductance is non-zero, which confirms the bulk transport data showing the material to remain metallic in this phase. For reference, we have included an equivalent measurement for pristine highly orientated pyrolytic graphite. The usual graphitic, semi-metallic behaviour is observed ( Fig. 6b ). Figure 6: Spectroscopic studies of stripe phase. ( a ) Numerically differentiated and averaged (60,000 spectra) spectroscopy, g (V) recorded at +800 mV, 50 pA set point on CaC 6 . ( b ) Numerically differentiated spectra recorded at the same set point on unintercalated graphite. ( c ) g ( q ,V) Fourier transform scanning tunnelling spectroscopic image at 0 mV. ( d–f ) g ( q ,V) Fourier intensity plotted as a function of energy for the stripe ( d , blue) and Superlattices A and B ( e , green and & f , yellow) spots marked in ( b ) respectively. These colours are chosen to match the respective directions marked in Figure 2 . Faint lines represent individual datasets, bold lines represent average. Red dotted line is the background intensity (already subtracted from all lines presented). Full size image The Fourier transform of the position-dependent conductivity allows us to access conductivity g ( q ,V) as a function of bias and q, the reciprocal space vector, conjugate to real-space position, allowing the association of electronic structure with specific q [28] . Figure 5c is a reciprocal-space conductivity image at 0 mV (that is, g( q x , q y ,0)). The bright spots match the reciprocal lattice positions for the stripe and superlattice, and do not change with bias; these features are dispersionless ( Supplementary Fig. S2 ). Superlattice A corresponds to the Ca symmetry direction that intersects the stripes in real-space (marked in green in Figure 2d,e ), Superlattice B corresponds to the Ca lattice direction that runs parallel to the stripes in real-space (marked in yellow in Fig. 2d ). The carbon reciprocal lattice spots are absent because of insufficient spatial resolution in the original CITS data. Figures 6d,e,f display the conductivities g ( q ,V) for the Stripe, Superlattice A and Superlattice B spots, respectively. g ( q ,V) for the Stripe spot exhibits two main peaks, separated by ~475 mV, around the Fermi level, where there is a minimum in the density of states. This analysis allows us to associate the gap shown in Figure 6a with the stripe q -vector. The broken Ca symmetry seen in Figure 3 is also reflected electronically. The true stripe-independent Ca contribution is seen for superlattice B ( Fig. 6f), and here the LDOS has a maximum near the Fermi level. However, Superlattice A ( Fig. 6e ) also has an extra component from a higher order stripe peak (3 q CDW ). Superlattice A has a greater contribution to the LDOS at negative bias than Superlattice B, which is consistent with the topographic images of Figure 5a,b (that is, the contrast between Ca atoms on and off the stripes is greater in negative bias imaging). CDWs have been suggested as a possible origin for a variety of anomalous long-range superlattices seen in graphite intercalation compounds and graphite by electron diffraction [29] and STM [30] , [31] . However, because of a lack of complementary electronic structure measurements, the authors of these reports were unable to rule out other effects, including Moiré patterns, observed in graphite [32] , electron standing waves, reported in various metals [33] , and surface reconstruction or lattice depletion [31] . It is therefore important to consider these phenomena when examining our data. In Figure 2, we demonstrate that the stripes coexist with the predicted carbon and Ca lattices. This precludes the possibility that the stripe phase is a surface reconstruction, that is, it results from a depletion or reorganization of the intercalant or carbon lattice. Second, a Moiré pattern could not lead to a gap in the LDOS. Finally, we have shown that the stripe period does not change with bias, thus ruling out electron standing waves and Friedel oscillations that are dispersing effects. However, our observations are consistent with a CDW. In fact, the direct association of a gap ( Fig. 6a ) with the stripe periodicity provides strong evidence that this is a CDW gap associated with the depletion of states around the Fermi level. The near-perfect inversion of contrast with bias polarity seen in Figure 4 is also characteristic of a true CDW [34] . The large gap size indicates a significant modification of the FS, but is consistent with that seen in other lamellar materials. For example, for NbSe 2 , 2Δ=68 meV with a transition temperature T CDW =33 K (ref. 9 ), which gives a ratio 2Δ/ k B T CDW =23.9 similar to that, 22.1, which we have measured for CaC 6 . We propose that the CDW mechanism is as follows: as the material is cooled, the negative thermal expansion of the graphene sheets flattens the planes, making an in-plane distortion of the Ca lattices between the graphene sheets (as observed) energetically favourable. The distortion is transverse and results in motion of charge on the graphene sheet immediately adjacent to the perturbed Ca atoms (hence the coincidence of the distorted atom with the stripe peak in positive bias and the stripe trough in negative bias) leading to the observed stripe phase. The hysteretic behaviour seen in magnetization is consistent with the one-way stripe decay observed in STM, indicating that the stringent flat, high-purity sample conditions required to maintain the CDW cannot be recovered if the sample transforms out of the CDW phase, where the sample crumples to raise the surface roughness as shown in Figure 3d . These requirements also explain why below the CDW transition, the sample behaves as a better metal than when it is in its normal high-temperature state ( Fig. 1 ). It is natural to ask whether FS nesting drives the CDW formation in CaC 6 . There are several reported FS, determined both experimentally [17] , [35] and theoretically [36] , [37] . These all exhibit the potential for nesting, namely that they have high symmetry, extended parallel portions of FS and significant density of states around the Fermi level. In spite of this, we find no nesting vectors matching the q -vector of the stripes. However, given various discrepancies between the candidate FS, such as missing or extra bands and differing values of charge transfer, together with the difficulties assigning the correct nesting vector for similar systems (for example, NbSe 2 (refs 34 , 38 , 39 ), we cannot discount this mechanism. We have presented the first measurement of the CDW state in the graphitic superconductor CaC 6 . The cleanliness and simplicity of this material compared with other layered superconductors makes it ideal for the study of the apparent ubiquity of CDWs and superconductivity in quasi-2D materials. Our data also represent a new demonstration of the remarkable rigidity of graphene—even with the very large density of mobile carriers donated by the Ca dopants, the large spectroscopic gap and other electronic manifestations of the CDW, we cannot detect any distortion of the carbon nuclei. This suggests that, within the graphene sheets, the dominant interaction is the electron–electron (e–e) repulsion and not the electron–phonon coupling that is clearly important for the Ca planes. The recent discoveries of the fractional quantum hall effect, and hints of an insulating Wigner crystal phase in graphene [15] , [40] also indicate that the e–e interaction has a more significant role than previously thought. Our results hold out the tantalizing possibility that eventually a graphene-based field-effect transistor might allow sufficient electron-doping (~1.5 eV shift of DOS in CaC 6 (ref. 17 ) typical maximum values in graphene through the field effect is currently ~0.8 eV (ref. 41 )) to induce a CDW and even superconductivity. Sample preparation The CaC 6 samples were fabricated from a highly orientated pyrolytic graphite platelet by the Lithium/Calcium alloy method [25] . The phase purity of the silver-coloured samples was confirmed by X-ray diffraction to be >99%. To protect the air-sensitive samples, they were fixed between a cleavage post and STM sample plate using conducting Ag-epoxy in an Argon atmosphere glove box (<0.1 p.p.m. O 2 , H 2 O) then transferred to the STM UHV chamber and cleaved at room temperature in situ immediately before scanning. For the transport and magnetization measurements, the samples were again manipulated and maintained in a strictly inert atmosphere of either argon or helium. STM methodology The STM experiments were carried out using an Omicron low-temperature STM at 78 K and UHV conditions (<10 −10 mbar). The STM tips were made from chemically etched tungsten wire. We found no spectroscopically stable or atomically resolved surfaces at room temperature; however, this may simply be due to instrumental limitations. Spectra taken during CITS measurements were recorded every 0.1 nm in a 10×10 nm 2 grid with a bias range of ±800 mV at a resolution of 8 mV (~ kT ). All STM data presented are unmanipulated, unless stated otherwise. STM images presented in Figures 2 , 3 and 4 were recorded on the same surface region (see Supplementary Fig. S3 for similar imaging on other surface regions). For Figure 3a the drift correction process is as follows: the image was sheared in the x -direction, rotated to bring the stripes parallel to the horizontal axis of the image, and then cropped. There was no warping of the lattice, as is sometimes the practice in drift correction of STM images and this image manipulation cannot produce the repeated (across multiple images) local transverse distortions reported. How to cite this article: Rahnejat, K.C. et al . Charge density waves in the graphene sheets of the superconductor CaC 6 . Nat. Commun. 2:558 doi: 10.1038/ncomms1574 (2011).